Centrin3 in trypanosomes maintains the stability of a flagellar inner-arm dynein for cell motility Centrin is a conserved component of centrioles in animals and basal bodies in flagellated organisms. It also associates with axonemal inner-arm dyneins and regulates cell motility, but the underlying mechanism remains elusive. In Trypanosoma brucei , three of the five centrins associate with the flagellar basal body, but no centrin has been found to regulate flagellar motility. Here we show that TbCentrin3 is a flagellar protein and knockdown of TbCentrin3 compromises cell motility. Tandem affinity purification followed by mass spectrometry identifies an inner-arm dynein, TbIAD5-1, as the TbCentrin3 partner, and knockdown of TbIAD5-1 causes similar cell motility defect. Further, we demonstrate the interdependence of TbCentrin3 and TbIAD5-1 for maintaining a stable complex in the flagellar axoneme. Together, these results identify the essential role of TbCentrin3 in cell motility by maintaining the stability of an inner-arm dynein in the flagellum, which may be shared by all the centrin-containing flagellated and ciliated organisms. Centrins are evolutionarily conserved calcium-binding proteins, which are ubiquitously found in eukaryotes and participate in a number of cellular processes, including centriole and basal body duplication [1] , [2] . Originally discovered in the flagellated green alga Chlamydomonas reinhardtii , centrin is located in the flagellum-anchoring basal apparatus and appears to constitute a component of a unique contractile filament system, which, consisting of rapid contractions and slow extensions, represents a novel cell motility mechanism distinct from the well-understood sliding mechanisms of actomyosin and dynein/microtubule [3] . In Chlamydomonas , the single centrin protein is localized to multiple distinct structures in the flagellar apparatus, including the flagellar basal body and the axoneme [4] , and is required for basal body duplication and segregation during cell division [1] . Centrin in the flagellar axoneme appears to associate with three inner-arm dynein heavy chains in Chlamydomonas flagellum [5] and in Tetrahymena cilium, where it regulates the motility of cilia in a calcium-dependent manner [6] . However, the precise mechanism by which centrin regulates flagellar and ciliary motility remains unknown. In Trypanosoma brucei , an early branching parasitic protozoan and the causative agent of human sleeping sickness, five centrins have been identified [7] , among which TbCentrin1 (aka TbCen3 (ref. 8 )), TbCentrin2 and TbCentrin4 (aka TbCen1 (ref. 9 )) are localized to the flagellar basal body. TbCentrin1 and TbCentrin2 are required for basal body duplication [7] . TbCentrin2 and TbCentrin4 are additionally enriched in the bilobe structure that is closely associated with the Golgi apparatus [7] , [9] , [10] . TbCentrin2 is essential for Golgi duplication [7] , whereas TbCentrin4 appears to regulate the abundance and function of TbCentrin2 on the bilobe [11] and also coordinates nuclear division with cell division through unknown mechanisms [10] . In another report, however, TbCentrin4 was found to be required for basal body segregation and cytokinesis [9] . Nevertheless, these studies demonstrated that at least three centrins, TbCentrin1, TbCentrin2 and TbCentrin4, associate with the flagellar basal body and regulate basal body duplication and segregation, and one of them, TbCentrin2, has an additional role in Golgi biogenesis [7] . Intriguingly, a recent study showed that TbCentrin2 also localizes to the flagellum [12] , but it appears that TbCentrin2 neither plays any essential role in flagellum biogenesis nor regulates flagellar motility [7] , [8] . Little is known about the subcellular localization and function of the two remaining centrins, TbCentrin3 (Tb927.10.8710) and TbCentrin5 (Tb927.11.13900), in T. brucei . Recently, TbCentrin3 was found in the proteome of a flagellum-associated complex that includes flagellum, basal body and bilobe [13] , but the precise subcellular localization and function of TbCentrin3 remain elusive. In this paper, we report that TbCentrin3 localizes to the flagellum and associates with one of the seven inner-arm dynein heavy chains. RNA interference (RNAi) of TbCentrin3 compromises cell motility and results in defective assembly of this inner-arm dynein in the flagellum and the accumulation of this dynein in the cytosol, where it is degraded by the 26S proteasome. Conversely, depletion of the TbCentrin3-interacting inner-arm dynein causes defective assembly of TbCentrin3 in the flagellum and degradation of TbCentrin3 in the cytosol. Our findings identify, for the first time, the essential role of TbCentrin3 in cell motility by maintaining the stability of an inner-arm dynein in the flagellar axoneme, which could be shared by all the centrin-containing flagellated and ciliated organisms. TbCentrin3 localizes to the flagellum To determine the subcellular localization of TbCentrin3, endogenous TbCentrin3 was tagged at the carboxy terminus with enhanced yellow fluorescence protein (EYFP). TbCentrin3::EYFP appeared to localize to the flagellum throughout the cell cycle in both the procyclic and bloodstream forms ( Fig. 1a,b ), indicating that TbCentrin3 associates with the flagellum and is expressed at all the cell cycle stages. To further confirm that TbCentrin3 is a flagellar protein, we prepared cytoskeleton and flagellar skeleton of both life cycle forms and found that TbCentrin3::EYFP was still associated with the flagellum ( Fig. 1c ). These results suggest that TbCentrin3 associates tightly with the flagellum, likely to be residing in the flagellar axoneme as its orthologue in Chlamydomonas . 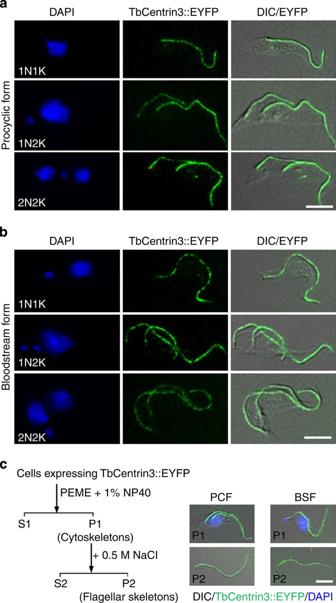Figure 1: TbCentrin3 is localized to the flagellum in both procyclic and bloodstream forms. Localization of TbCentrin3::EYFP in procyclic form (a) and bloodstream form (b). Cells expressing endogenously tagged TbCentrin3::EYFP were treated with PEME buffer containing 1% NP-40, counterstained with DAPI and visualized under a fluorescence microscope.Scale bar, 5 μm. (c). TbCentrin3 associates tightly with the flagellum in both the procyclic and bloodstream forms. Cells expressing EYFP-tagged TbCentrin3 were treated with PEME buffer containing 1% NP-40 to prepare cytoskeleton (P1). The cytoskeleton was further treated with PMN buffer containing 1% NP-40 and 500 mM NaCl to prepare flagellar skeleton (P2). The cytoskeleton (P1) and flagellar skeleton (P2) were visualized under the fluorescence microscope. Scale bar, 5 μm. Figure 1: TbCentrin3 is localized to the flagellum in both procyclic and bloodstream forms. Localization of TbCentrin3::EYFP in procyclic form ( a ) and bloodstream form ( b ). Cells expressing endogenously tagged TbCentrin3::EYFP were treated with PEME buffer containing 1% NP-40, counterstained with DAPI and visualized under a fluorescence microscope.Scale bar, 5 μm. ( c ). TbCentrin3 associates tightly with the flagellum in both the procyclic and bloodstream forms. Cells expressing EYFP-tagged TbCentrin3 were treated with PEME buffer containing 1% NP-40 to prepare cytoskeleton (P1). The cytoskeleton was further treated with PMN buffer containing 1% NP-40 and 500 mM NaCl to prepare flagellar skeleton (P2). The cytoskeleton (P1) and flagellar skeleton (P2) were visualized under the fluorescence microscope. Scale bar, 5 μm. Full size image TbCentrin3 RNAi causes motility defect in procyclic form The localization of TbCentrin3 in the flagellum implies that it may play important roles in the flagellum. To understand the function of TbCentrin3, RNAi was performed in the procyclic form. Quantitative reverse transcription–PCR showed that the mRNA level of TbCentrin3 in the RNAi cells was decreased to ~10% of the non-induced control cells after tetracycline induction for 2 days ( Fig. 2a ). Western blotting showed that TbCentrin3 protein, which was endogenously tagged with a PTP ( P rotein A- T EV- P rotein C) epitope [14] , was also significantly reduced on RNAi induction ( Fig. 2b ). Depletion of TbCentrin3 only slightly slowed down cell growth ( Fig. 2c ). However, these RNAi-induced cells appeared to lose motility in the culture medium as observed under a light microscope. Loss of cell motility occurred at as early as day 1 of RNAi induction, and at day 3 of RNAi almost all cells lost motility. To confirm the motility defect, we carried out two experiments, sedimentation assay and motility tracing, to quantitatively characterize the motility of the non-induced control and TbCentrin3 RNAi cells at day 3 of RNAi induction. Sedimentation assay showed that TbCentrin3 RNAi cells were precipitated at the bottom of the cuvette as reflected by the low optical density ( Fig. 2d ). Moreover, motility traces showed that TbCentrin3 RNAi cells were only able to move a very short distance as compared with the non-induced control cells ( Fig. 2e, f ). Notably, the flagellum of the RNAi cells appeared to be still capable of beating, but the cells were not able to move a long distance, thus remaining at one location or just spinning and tumbling ( Supplementary Movie 1 ), which was in striking contrast to the non-induced control cells that travelled very quickly from one location to another ( Supplementary Movie 2 ). These results suggest that TbCentrin3 is required for directional cell motility in procyclic trypanosomes. The motility defect apparently was not due to a gross structural alteration of the flagellum, because electron microscopic analysis of the flagellum of TbCentrin3 RNAi cells showed that the axoneme 9+2 microtubules and the paraflagellar rod (PFR), an elaborate extra-axoneme structure, are both unaffected ( Supplementary Fig. 1 ). Similarly, RNAi of another inner-arm dynein, DNAH10, in procyclic trypanosomes also caused severe motility defect, but did not disrupt axoneme structure [15] , [16] . 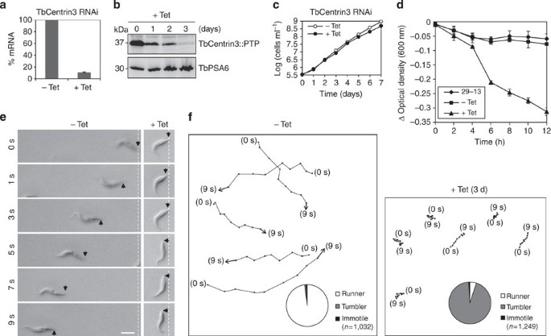Figure 2: RNAi of TbCentrin3 in procyclic trypanosomes impairs cell motility. (a) TbCentrin3 mRNA level in non-induced control cells and RNAi cells detected by quantitative reverse transcription–PCR. Three independent experiments were carried out and the error bars represent s.d. (b) TbCentrin3::PTP protein level in control and RNAi cells detected by western blotting with anti-Protein A antibody. Level of TbPSA6, the α6 subunit of the 26S proteasome, was included as the loading control. (c) RNAi of TbCentrin3 slowed down cell proliferation. (d) Sedimentation assays to monitor cell motility. The parental 29-13 strain, the non-induced control and RNAi cells after tetracycline induction for 3 days were incubated in cuvettes, and the cell density (optical density) was determined and plotted against the time of incubation (hours). Three independent experiments were carried out and the error bars represent s.d. (e,f) Tracing the motility of non-induced control cells and TbCentrin3 RNAi cells (day 3) by video microscopy. Black arrows indicate the posterior tip of the cells, and the white dashed lines show the posterior of cells at the start of time-lapse video microscopy. Scale bar, 10 μm. Pie charts inserted infshow the percentage of cells scored as runner (white), tumbler (grey) or immotile (black) in non-induced control and TbCentrin3 RNAi cells.n, number of cells counted. Figure 2: RNAi of TbCentrin3 in procyclic trypanosomes impairs cell motility. ( a ) TbCentrin3 mRNA level in non-induced control cells and RNAi cells detected by quantitative reverse transcription–PCR. Three independent experiments were carried out and the error bars represent s.d. ( b ) TbCentrin3::PTP protein level in control and RNAi cells detected by western blotting with anti-Protein A antibody. Level of TbPSA6, the α6 subunit of the 26S proteasome, was included as the loading control. ( c ) RNAi of TbCentrin3 slowed down cell proliferation. ( d ) Sedimentation assays to monitor cell motility. The parental 29-13 strain, the non-induced control and RNAi cells after tetracycline induction for 3 days were incubated in cuvettes, and the cell density (optical density) was determined and plotted against the time of incubation (hours). Three independent experiments were carried out and the error bars represent s.d. ( e , f ) Tracing the motility of non-induced control cells and TbCentrin3 RNAi cells (day 3) by video microscopy. Black arrows indicate the posterior tip of the cells, and the white dashed lines show the posterior of cells at the start of time-lapse video microscopy. Scale bar, 10 μm. Pie charts inserted in f show the percentage of cells scored as runner (white), tumbler (grey) or immotile (black) in non-induced control and TbCentrin3 RNAi cells. n , number of cells counted. Full size image TbCentrin3 associates with inner-arm dynein TbIAD5-1 To identify TbCentrin3-associated protein(s) in the flagellum, we carried out tandem affinity purification. TbCentrin3 was in situ tagged at the amino terminus with the PTP tag at one of its two endogenous loci in the procyclic form. Western blotting with anti-Protein C antibody detected a single protein band of the expected molecular mass ( Fig. 3a ), and immunostaining with anti-Protein A antibody confirmed that PTP-tagged TbCentrin3 was correctly localized to the flagellum (see Fig. 6a below). As TbCentrin3 is a flagellar protein ( Fig. 1 ), we prepared cell lysate by thorough sonication, through which the flagellum structure is known to be disrupted and flagellum-associated protein complexes can be readily purified by immunoprecipitation (IP) [17] . The crude lysate was then applied to tandem affinity purification [14] . The final eluate was separated by SDS–polyacrylamide gel electrophoresis (SDS–PAGE) and stained with silver solution. Several distinct protein bands were detected ( Fig. 3b ). The biggest protein band exhibited a molecular mass way over 250 kDa ( Fig. 3b ), and liquid chromatography–tandem mass spectrometry (LC-MS/MS) showed that this band represented Tb927.7.920, which encodes a putative inner-arm dynein with a predicted molecular mass of 465 kDa and is one of the two IAD5-family dyneins that share an overall sequence identify of 33.2% [18] . We named this dynein TbIAD5-1. The other protein bands between 50–150 kDa were degradation products of TbIAD5-1. 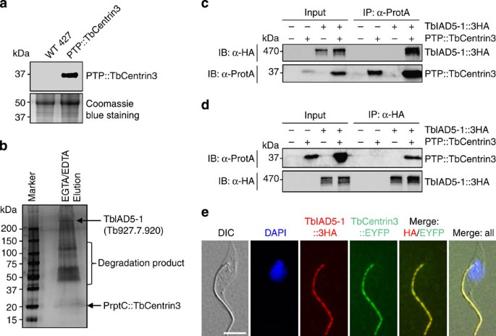Figure 3: TbCentrin3 associates with TbIAD5-1, an inner-arm dynein heavy chain. (a) Western blotting with anti-Protein C antibody to detect the endogenously PTP-tagged TbCentrin3. (b) SDS–PAGE analysis of TbCentrin3-associated proteins. Shown is the final EGTA/EDTA elution of TbCentrin3 PTP purification, which was silver stained. (c) IP of PTP::TbCentrin3 to precipitate TbIAD5-1::3HA from trypanosome lysate. PTP::TbCentrin3 was detected by anti-Protein A pAb (anti-ProtA) and TbIAD5-1::3HA was detected by anti-HA mAb. (d) IP of TbIAD5-1::3HA to pull down PTP::TbCentrin3 from trypanosome lysate. (e) Co-localization of TbCentrin3 and TbIAD5-1 in procyclic trypanosomes. Endogenous TbCentrin3 was tagged with EYFP and endogenous TbIAD5-1 was tagged with a triple HA epitope in the same cell line. Cells were immunostained with anti-HA antibody and Cy3-conjugated anti-mouse IgG and counterstained with DAPI. Scale bar, 5 μm. Figure 3: TbCentrin3 associates with TbIAD5-1, an inner-arm dynein heavy chain. ( a ) Western blotting with anti-Protein C antibody to detect the endogenously PTP-tagged TbCentrin3. ( b ) SDS–PAGE analysis of TbCentrin3-associated proteins. Shown is the final EGTA/EDTA elution of TbCentrin3 PTP purification, which was silver stained. ( c ) IP of PTP::TbCentrin3 to precipitate TbIAD5-1::3HA from trypanosome lysate. PTP::TbCentrin3 was detected by anti-Protein A pAb (anti-ProtA) and TbIAD5-1::3HA was detected by anti-HA mAb. ( d ) IP of TbIAD5-1::3HA to pull down PTP::TbCentrin3 from trypanosome lysate. ( e ) Co-localization of TbCentrin3 and TbIAD5-1 in procyclic trypanosomes. Endogenous TbCentrin3 was tagged with EYFP and endogenous TbIAD5-1 was tagged with a triple HA epitope in the same cell line. Cells were immunostained with anti-HA antibody and Cy3-conjugated anti-mouse IgG and counterstained with DAPI. Scale bar, 5 μm. Full size image Figure 6: Effect of TbIAD5-1 knockdown on the localization and stability of TbCentrin3. ( a ). 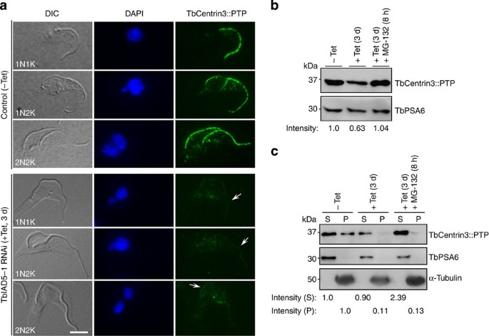Figure 6: Effect of TbIAD5-1 knockdown on the localization and stability of TbCentrin3. (a). TbIAD5-1 RNAi on TbCentrin3 localization to the flagellum. Endogenous TbCentrin3 was tagged with a C-terminal PTP epitope in cells harbouring the TbIAD5-1 RNAi construct. RNAi was induced by tetracycline for 3 days and cytoskeleton was prepared for immunostaining with anti-Protein A pAb and fluorescein isothiocyanate (FITC)-conjugated anti-rabbit IgG. Arrows indicate the weak TbCentrin3::PTP signal at the flagellum on TbIAD5-1 RNAi.Scale bar, 5 μm. (b) Effect of TbIAD5-1 RNAi on TbCentrin3 protein stability. Crude lysate was analysed by western blotting with anti-Protein A pAb to detect PTP-tagged TbCentrin3. Level of TbPSA6 served as the loading control. The intensity of protein bands was determined with ImageJ and TbCentrin3 level was normalized with the loading control. (c) Effect of TbIAD5-1 RNAi on TbCentrin3 protein stability in cytosolic and the cytoskeletal fractions. Preparation of cytosolic and cytoskeletal fractions was carried out essentially as described inFig. 5. TbCentrin3::PTP was detected by anti-Protein A pAb. α-Tubulin and TbPSA6 served as the control for cytoskeletal and cytosolic proteins, respectively. The intensity of protein bands was determined with ImageJ and normalized against the loading control. At least three repeats were performed. TbIAD5-1 RNAi on TbCentrin3 localization to the flagellum. Endogenous TbCentrin3 was tagged with a C-terminal PTP epitope in cells harbouring the TbIAD5-1 RNAi construct. RNAi was induced by tetracycline for 3 days and cytoskeleton was prepared for immunostaining with anti-Protein A pAb and fluorescein isothiocyanate (FITC)-conjugated anti-rabbit IgG. Arrows indicate the weak TbCentrin3::PTP signal at the flagellum on TbIAD5-1 RNAi.Scale bar, 5 μm. ( b ) Effect of TbIAD5-1 RNAi on TbCentrin3 protein stability. Crude lysate was analysed by western blotting with anti-Protein A pAb to detect PTP-tagged TbCentrin3. Level of TbPSA6 served as the loading control. The intensity of protein bands was determined with ImageJ and TbCentrin3 level was normalized with the loading control. ( c ) Effect of TbIAD5-1 RNAi on TbCentrin3 protein stability in cytosolic and the cytoskeletal fractions. Preparation of cytosolic and cytoskeletal fractions was carried out essentially as described in Fig. 5 . TbCentrin3::PTP was detected by anti-Protein A pAb. α-Tubulin and TbPSA6 served as the control for cytoskeletal and cytosolic proteins, respectively. The intensity of protein bands was determined with ImageJ and normalized against the loading control. At least three repeats were performed. Full size image To confirm the in vivo interaction between TbCentrin3 and TbIAD5-1, we carried out co-IP. Endogenously PTP-tagged TbCentrin3 and triple haemagglutinin (HA)-tagged TbIAD5-1 were co-expressed in the same cell line. IP of TbCentrin3::PTP was capable of pulling down TbIAD5-1::3HA from the cell lysate prepared by sonication ( Fig. 3c ). Reciprocal IP with anti-HA antibody for precipitation of TbIAD5-1::3HA was also able to pull down TbCentrin3::PTP from trypanosome cell lysate ( Fig. 3d ). These results further confirm that TbCentrin3 indeed interacts with TbIAD5-1 in vivo and suggest that TbCentrin3 is a component of an inner-arm dynein complex in trypanosomes. To determine the subcellular localization of TbIAD5-1 as well as to examine whether it co-localizes with TbCentrin3, we tagged the endogenous TbIAD5-1 with a C-terminal triple HA epitope in the procyclic cell line expressing endogenously EYFP-tagged TbCentrin3. In all the cells examined, TbIAD5-1::3HA was found in the flagellum throughout the cell cycle and co-localized with TbCentrin3::EYFP ( Fig. 3e and data not shown). Given that TbCentrin3 and TbIAD5-1 interact in vivo ( Fig. 3b–d ), these observations suggest that the two proteins form a complex in the flagellum. TbIAD5-1 RNAi leads to motility defect in the procyclic form To investigate the function of TbIAD5-1, RNAi was carried out in the procyclic form. After RNAi induction for 2 days, TbIAD5-1 mRNA was decreased to ~30% of that in the non-induced control cells as measured by quantitative reverse transcription–PCR ( Fig. 4a ). The protein level of TbIAD5-1, which was endogenously tagged with a triple HA epitope, was gradually decreased from the first day of RNAi induction and reached the lowest level after 3 days of RNAi, but the protein was not completely depleted ( Fig. 4b ). This significant downregulation of TbIAD5-1 in the procyclic form only slightly slowed down cell growth ( Fig. 4c ), similar to the growth defect of TbCentrin3 RNAi cells ( Fig. 2c ). Similar to TbCentrin3 RNAi, TbIAD5-1 RNAi also caused severe defect in cell motility as demonstrated by sedimentation assay ( Fig. 4d ), motility tracing ( Fig. 4e,f ) and time-lapse video microscopy ( Supplementary Movie 3 ). Although the flagella of the TbIAD5-1 RNAi cells were still capable of beating, the RNAi cells apparently lost directional motility and, instead, were just spinning and tumbling, remaining primarily at one location, or only travelled a short distance ( Fig. 4e,f and Supplementary Movie 3 ). In contrast, the non-induced control cells were able to travel a long distance in a short time under the same experimental conditions ( Fig. 4e,f and Supplementary Movie 4 ). The motility defect caused by TbIAD5-1 RNAi was very similar to that caused by TbCentrin3 RNAi. Given that the two proteins interact in vivo in the flagellum ( Fig. 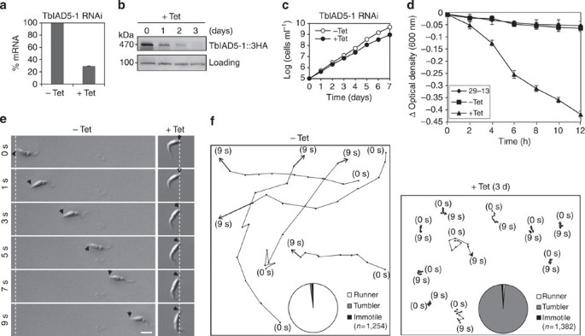3 ), TbCentrin3 apparently plays an essential role in the TbIAD5-1 complex. Figure 4: RNAi of TbIAD5-1 in the procyclic form causes defects in cell motility. (a) TbIAD5-1 mRNA level in non-induced control and RNAi-induced cells detected by quantitative reverse transcription–PCR. Three independent experiments were carried out and the error bars represent s.d. (b) TbIAD5-1::3HA protein level in non-induced control and RNAi cells detected by western blotting with anti-HA antibody. Level of a nonspecific protein cross-reacted with anti-HA antibody served as the loading control. (c) RNAi of TbIAD5-1 slowed down cell proliferation. (d) Sedimentation assays to monitor cell motility. The parental 29-13 strain, the non-induced control and TbIAD5-1 RNAi cells after tetracycline induction for 3 days were incubated in cuvettes and cell density (optical density) was determined and plotted against the time of incubation (h). Three independent experiments were carried out and the error bars represent s.d. (e,f) Tracing the motility of non-induced control cells and TbIAD5-1 RNAi cells (day 3) by video microscopy. Black arrows indicate the posterior tip of the cells, and the white dashed lines show the posterior of cells at the start of time-lapse video microscopy. Scale bar, 10 μm. Pie charts inserted infshow the percentage of cells scored as runner (white), tumbler (grey) or immotile (black) in non-induced control and TbIAD5-1 RNAi cells.n, number of cells counted. Figure 4: RNAi of TbIAD5-1 in the procyclic form causes defects in cell motility. ( a ) TbIAD5-1 mRNA level in non-induced control and RNAi-induced cells detected by quantitative reverse transcription–PCR. Three independent experiments were carried out and the error bars represent s.d. ( b ) TbIAD5-1::3HA protein level in non-induced control and RNAi cells detected by western blotting with anti-HA antibody. Level of a nonspecific protein cross-reacted with anti-HA antibody served as the loading control. ( c ) RNAi of TbIAD5-1 slowed down cell proliferation. ( d ) Sedimentation assays to monitor cell motility. The parental 29-13 strain, the non-induced control and TbIAD5-1 RNAi cells after tetracycline induction for 3 days were incubated in cuvettes and cell density (optical density) was determined and plotted against the time of incubation (h). Three independent experiments were carried out and the error bars represent s.d. ( e , f ) Tracing the motility of non-induced control cells and TbIAD5-1 RNAi cells (day 3) by video microscopy. Black arrows indicate the posterior tip of the cells, and the white dashed lines show the posterior of cells at the start of time-lapse video microscopy. Scale bar, 10 μm. Pie charts inserted in f show the percentage of cells scored as runner (white), tumbler (grey) or immotile (black) in non-induced control and TbIAD5-1 RNAi cells. n , number of cells counted. Full size image TbCentrin3 is required for assembly of TbIAD5-1 We tested whether TbCentrin3 knockdown affects the localization of TbIAD5-1 to the flagellum. Immunostaining of paraformaldehyde-fixed intact cells with anti-HA antibody was not able to detect TbIAD5-1::3HA, likely to be because the antibody could not access the flagellum in intact cells. We therefore prepared detergent-extracted cytoskeleton for immunostaining. In the non-induced control cells, TbIAD5-1 was found uniformly distributed throughout the length of both the new and old flagella ( Fig. 5a ). Strikingly, TbIAD5-1 appeared to be gradually depleted from the flagellum on TbCentrin3 RNAi ( Fig. 5a ). The depletion of TbIAD5-1 occurred as early as 16 h after TbCentrin3 RNAi and appeared to occur predominantly in the new flagellum in ~85% of the 1N2K and 2N2K cells ( Supplementary Fig. 2A and Fig. 5b , 1N2K and 2N2K, 16 h, weak/strong TbIAD5-1 signal), although ~10% of the 1N2K cells contained weak TbIAD5-1 signal in both the new and old flagella ( Supplementary Fig. 2A and Fig. 5b , 1N2K, 16 h, weak/weak TbIAD5-1 signal). Moreover, ~50% of the 1N1K cells also contained weak TbIAD5-1 signal in the single flagellum ( Supplementary Fig. 2A , square bracket, and Fig. 5b , 1N1K, 16 h), and in some 1N2K and 2N2K cells TbIAD5-1 appeared to be depleted from the tip of the old flagellum ( Supplementary Fig. 2A , small square brackets). After TbCentrin3 RNAi for 24 h more cells lost TbIAD5-1 from the flagellum ( Fig. 5a,b , 24 h), and after TbCentrin3 RNAi for 72 h all the cells (1N1K, 1N2K and 2N2K) contained weak TbIAD5-1 signal throughout the flagella ( Supplementary Fig. 2B and Fig. 5b ), with the proximal portion of both the new and old flagella containing slightly reduced TbIAD5-1 signal ( Supplementary Fig. 2B , arrows) and the remaining portion of the flagella containing significantly reduced TbIAD5-1 signal. 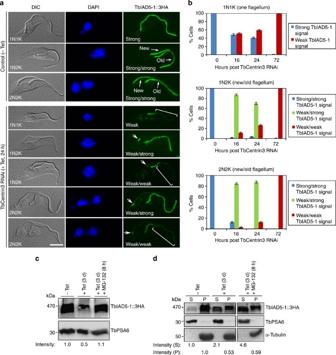These results suggest that RNAi of TbCentrin3 led to failure in assembling the TbIAD5-1 complex in the new flagellum and probably also caused disassembly of the TbIAD5-1 complex from the tip of the old flagellum. Figure 5: Effect of TbCentrin3 knockdown on the localization and stability of TbIAD5-1. (a) TbCentrin3 RNAi on TbIAD5-1 localization to the flagellum. Endogenous TbIAD5-1 was tagged with a C-terminal triple HA epitope in cells harbouring the TbCentrin3 stem-loop RNAi construct. TbCentrin3 RNAi was induced by tetracycline for 24 h and cytoskeleton was prepared for immunostaining with fluorescein isothiocyanate (FITC)-conjugated anti-HA mAb. New and old flagella are indicated. Arrows in TbCentrin3 RNAi cells indicate the TbIAD5-1 signal at the proximal portion of the flagellum. The square brackets outline the portion of flagellum where TbIAD5-1 signal was reduced. For 1N1K cells, strong or weak signal refers to the TbIAD5-1 signal on the single flagellum. For 1N2K and 2N2K cells, strong/strong signal: strong TbIAD5-1 signal on both new and old flagella; weak/strong signal: weak TbIAD5-1 signal on the new flagellum and strong TbIAD5-1 signal on the old flagellum; weak/weak signal: weak TbIAD5-1 signal on both new and old flagella.Scale bar, 5 μm. (b) Quantification of control and TbCentrin3 RNAi cells with different intensity of TbIAD5-1 fluorescence signal. Data are presented as the mean percentage±s.d. of ~300 cells counted from each of the three independent experiments. All cells from the captured images were counted. (c) Effect of TbCentrin3 RNAi on TbIAD5-1 stability. Crude lysate was analysed by western blotting with anti-HA mAb to detect 3HA-tagged TbIAD5-1. TbPSA6 level served as the loading control. The intensity of the protein bands was determined with ImageJ and TbIAD5-1 level was normalized with the loading control. (d) Effect of TbCentrin3 RNAi on TbIAD5-1 protein stability in cytosolic and the cytoskeletal fractions. Non-induced control and TbCentrin3 RNAi cells were lysed in PEME buffer containing 1% NP-40 for cytoskeleton preparation. The soluble cytosolic fraction (S) and cytoskeletal pellet fraction (P) were separated by centrifugation, loaded onto a SDS–PAGE gel and transferred onto a polyvinylidene difluoride membrane for western blotting with anti-HA antibody to detect TbIAD5-1::3HA. The cytosolic fraction was detected by anti-TbPSA6, whereas the cytoskeletal fraction was detected by anti-α-tubulin. The intensity of the protein bands was determined with ImageJ as described above. At least three repeats were carried out. Figure 5: Effect of TbCentrin3 knockdown on the localization and stability of TbIAD5-1. ( a ) TbCentrin3 RNAi on TbIAD5-1 localization to the flagellum. Endogenous TbIAD5-1 was tagged with a C-terminal triple HA epitope in cells harbouring the TbCentrin3 stem-loop RNAi construct. TbCentrin3 RNAi was induced by tetracycline for 24 h and cytoskeleton was prepared for immunostaining with fluorescein isothiocyanate (FITC)-conjugated anti-HA mAb. New and old flagella are indicated. Arrows in TbCentrin3 RNAi cells indicate the TbIAD5-1 signal at the proximal portion of the flagellum. The square brackets outline the portion of flagellum where TbIAD5-1 signal was reduced. For 1N1K cells, strong or weak signal refers to the TbIAD5-1 signal on the single flagellum. For 1N2K and 2N2K cells, strong/strong signal: strong TbIAD5-1 signal on both new and old flagella; weak/strong signal: weak TbIAD5-1 signal on the new flagellum and strong TbIAD5-1 signal on the old flagellum; weak/weak signal: weak TbIAD5-1 signal on both new and old flagella.Scale bar, 5 μm. ( b ) Quantification of control and TbCentrin3 RNAi cells with different intensity of TbIAD5-1 fluorescence signal. Data are presented as the mean percentage±s.d. of ~300 cells counted from each of the three independent experiments. All cells from the captured images were counted. ( c ) Effect of TbCentrin3 RNAi on TbIAD5-1 stability. Crude lysate was analysed by western blotting with anti-HA mAb to detect 3HA-tagged TbIAD5-1. TbPSA6 level served as the loading control. The intensity of the protein bands was determined with ImageJ and TbIAD5-1 level was normalized with the loading control. ( d ) Effect of TbCentrin3 RNAi on TbIAD5-1 protein stability in cytosolic and the cytoskeletal fractions. Non-induced control and TbCentrin3 RNAi cells were lysed in PEME buffer containing 1% NP-40 for cytoskeleton preparation. The soluble cytosolic fraction (S) and cytoskeletal pellet fraction (P) were separated by centrifugation, loaded onto a SDS–PAGE gel and transferred onto a polyvinylidene difluoride membrane for western blotting with anti-HA antibody to detect TbIAD5-1::3HA. The cytosolic fraction was detected by anti-TbPSA6, whereas the cytoskeletal fraction was detected by anti-α-tubulin. The intensity of the protein bands was determined with ImageJ as described above. At least three repeats were carried out. Full size image To rule out a general effect of TbCentrin3 depletion on the inner-arm dyneins in the flagellum, we investigated the effect of TbCentrin3 RNAi on two other inner-arm dyneins, TbIAD5-2 (Tb927.11.11220) and TbIAD3 (Tb927.2.5270) [18] . The results showed that RNAi of TbCentrin3 did not abrogate the localization of TbIAD5-2 and TbIAD3 to the flagellum ( Supplementary Fig. 3 ), suggesting a specific effect of TbCentrin3 knockdown on TbIAD5-1 in the flagellum. The depletion of TbIAD5-1 from the flagellum in TbCentrin3 RNAi cells may be either due to the displacement of TbIAD5-1 from the flagellum to the cytosol, where TbIAD5-1 became soluble and was washed off when preparing detergent-extracted cytoskeleton and hence was not detected by immunofluorescence microscopy, or due to the failure in assembly of TbIAD5-1 in the flagellar axoneme, thus leaving TbIAD5-1 in the cytosol, or attributed to the in situ degradation of TbIAD5-1 in the flagellum. If the first two hypotheses are correct, then TbIAD5-1 protein level in crude cell lysate should not change on TbCentrin3 RNAi. To test this assumption, we carried out western blotting on whole-cell lysate, which showed that after TbCentrin3 RNAi for 3 days TbIAD5-1 protein level was reduced to ~50% of the control level ( Fig. 5c ). However, when the proteasome inhibitor MG-132 was added to TbCentrin3 RNAi cells, TbIAD5-1 was stabilized ( Fig. 5c ). These results suggest that TbIAD5-1 became unstable when TbCentrin3 was depleted. To further investigate whether TbIAD5-1 was degraded in the flagellum or in the cytosol, we prepared detergent-extracted cytoskeletal (pellet) fraction and cytosolic (soluble) fraction for western blotting, and the results showed that TbIAD5-1 level in the cytoskeletal fraction was decreased to ~50% of the control level after TbCentrin3 RNAi, but TbIAD5-1 level in the cytosolic fraction was instead increased about onefold in TbCentrin3 RNAi cells ( Fig. 5d ). Moreover, treatment of TbCentrin3 RNAi cells with MG-132 resulted in about onefold increase of TbIAD5-1 in the cytosolic fraction as compared with the TbIAD5-1 level in TbCentrin3 RNAi cells without MG-132 treatment ( Fig. 5d ). In contrast, TbIAD5-1 in the cytoskeletal fraction after MG-132 treatment was only slightly increased as compared with that in TbCentrin3 RNAi cells ( Fig. 5d ). These results suggest that TbIAD5-1 was degraded in the cytosol by the 26S proteasome. As TbIAD5-1 is an inner-arm dynein playing an essential role in flagellar motility ( Fig. 4 ), the motility defect of TbCentrin3 RNAi cells probably is attributed to the failure in assembly of TbIAD5-1 in the flagellar axoneme. These observations suggest an essential role of TbCentrin3 in cell motility by maintaining the stability of the inner-arm dynein TbIAD5-1 in the flagellar axoneme. TbIAD5-1 is required for assembly of TbCentrin3 We next examined the effect of TbIAD5-1 RNAi on TbCentrin3 by tagging the endogenous TbCentrin3 with a PTP epitope in the TbIAD5-1 RNAi cell line. Immunofluorescence microscopy showed that TbCentrin3 was evenly distributed throughout the length of the new and old flagella in the non-induced control cells ( Fig. 6a ). However, on TbIAD5-1 RNAi induction TbCentrin3 signal in the flagellum was significantly decreased ( Fig. 6a , arrows), suggesting that TbIAD5-1 is required for maintaining TbCentrin3 in the flagellum. Unlike TbIAD5-1, which remained at the proximal part of the flagellum on TbCentrin3 RNAi ( Fig. 5a ), TbCentrin3 appeared to be evenly depleted from the flagellum ( Fig. 6a ). The mechanism behind this difference is not known. Nevertheless, this result suggests that TbIAD5-1 is also required for assembly of TbCentrin3 to the flagellar axoneme. We next asked whether TbCentrin3 was degraded in the absence of TbIAD5-1. After TbIAD5-1 RNAi for 3 days, TbCentrin3 level was reduced to ~63% of the control level and MG-132 treatment of the RNAi cells resulted in stabilization of TbCentrin3 ( Fig. 6b ), suggesting that TbCentrin3 was degraded when TbIAD5-1 was depleted. To further investigate whether TbCentrin3 was degraded in situ in the flagellum or in the cytosol, we prepared cytosolic and cytoskeletal fractions for western blotting and the results showed that on TbIAD5-1 RNAi the level of TbCentrin3 in the cytoskeletal fraction was reduced to ~10% of the control level ( Fig. 6c ). In the cytosolic fraction, TbCentrin3 level was slightly reduced to ~90% of the control level ( Fig. 6c ). When MG-132 was added to the RNAi cells, TbCentrin3 level in the cytoskeletal fraction was similar to that in the RNAi cells without MG-132 treatment, whereas in the cytosolic fraction it was increased to about 2.4-fold of the control level ( Fig. 6c ), indicating that TbCentrin3 was stabilized in the cytosol. These results suggest that in the absence of TbIAD5-1, TbCentrin3 either was not assembled to the flagellar axoneme, thus remaining in the cytosol, or was released from the flagellum to the cytosol. In either case, TbCentrin3 apparently was degraded by the 26S proteasome ( Fig. 6c ). Intriguingly, the effect of TbIAD5-1 depletion on TbCentrin3 stability and assembly to the flagellum resembles that of TbCentrin3 depletion on TbIAD5-1 stability and assembly ( Fig. 5c ), suggesting the interdependence of the two proteins for maintaining a stable complex in the flagellar axoneme. The presence of five centrin-like proteins in T. brucei , a unicellular flagellated eukaryote, argues that each of the five centrins could perform specialized functions, which in other flagellated organisms such as Chlamydomonas are likely to be executed by the single centrin. Indeed, at least three T. brucei centrins, TbCentrin1, TbCentrin2 and TbCentrin4, associate with the flagellar basal body. TbCentrin1 and TbCentrin2 regulate basal body duplication/segregation [7] , [9] , and TbCentrin2 and TbCentrin4 also are enriched at the bilobe structure, and regulate Golgi biogenesis and coordinate cell and nuclear division, respectively [7] , [10] . TbCentrin2 was recently found in the flagellum in addition to the basal body and the bilobe structure [12] , and is regulated by the Polo-like kinase TbPLK for flagellum attachment zone filament assembly [19] . However, localization of TbCentrin2 to the flagellum was not observed in another study [7] . The discrepancy between the two studies could be that the two studies used anti-TbCentrin2 antibody and EYFP-tagged TbCentrin2 for localization, respectively. Nevertheless, no matter whether TbCentrin2 is localized to the flagellum, its primary function appears to control basal body duplication/segregation and Golgi duplication with little involvement in cell motility and flagellum biogenesis [7] , [8] . Unlike TbCentrin2, the primary function of TbCentrin3 is to control cell motility ( Fig. 2 and Supplementary Movie 1 ). Therefore, if TbCentrin2 is indeed a flagellar protein and plays a role in the flagellum, it is highly likely to be that TbCentrin2 and TbCentrin3 function in distinct pathways in the flagellum. Based on the previous reports and our current finding, it is fairly clear that the five centrins in T. brucei play specialized roles, with TbCentrin1 and TbCentrin2 in basal body duplication, TbCentrin2 additionally in bilobe duplication and Golgi biogenesis, TbCentrin4 in coordination of cell and nuclear division, and TbCentrin3 in cell motility. Other than TbCentrin2 and TbCentrin3, the other three centrins were also found in the flagellar proteome previously [20] , [21] . Therefore, it appears that multiple centrins associate with flagellum and flagellum-associated structures. However, TbCentrin1 and TbCentrin4 apparently are not involved in flagellar motility [7] , [10] . It would be interesting to investigate whether TbCentrin5 has a role in flagellar motility. The fact that centrins in trypanosomes play specialized functions offers unique advantages for dissecting the role of centrins in the respective cellular processes. RNAi of TbCentrin3 in the procyclic form of T. brucei clearly compromises directional cell motility, but does not paralyse the cell ( Fig. 2 and Supplementary Movie 1 ). The RNAi cells still possess flagellar beating capability, but they are unable to move a long distance. Instead, the RNAi cells just spin and tumble, remaining mostly at one location, or occasionally move backward ( Fig. 2e,f and Supplementary Movie 1 ). Our biochemical purification of the inner-arm dynein TbIAD5-1 as the partner of TbCentrin3 ( Fig. 3 ) suggests that TbCentrin3 is a component of an inner-arm dynein complex in the flagellar axoneme. RNAi of TbIAD5-1 resulted in motility defects similar to that caused by TbCentrin3 RNAi ( Fig. 4 ), thus providing compelling evidence that TbCentrin3 functions as an essential component of this inner-arm dynein complex. Given that centrins in Chlamydomonas and Tetrahymena associate with the inner-arm dyneins [6] , [22] , [23] , the identification of TbCentrin3 as a light chain of an inner-arm dynein complex in T. brucei and the involvement of TbCentrin3 in cell motility suggest the conserved role of centrin in cell motility in flagellated and ciliated organisms. Among the seven inner-arm dyneins in trypanosomes [18] , only TbIAD5-1 was co-precipitated with TbCentrin3 ( Fig. 3 ), in striking contrast to Chlamydomonas where three of the eight inner-arm dyneins interact with centrin [23] , [24] . These three inner-arm dynein complexes also contain actin [23] , [24] , but our tandem affinity purification using either TbCentrin3 or TbIAD5-1 as the bait did not precipitate actin ( Fig. 3 and data not shown). Whether actin is a component of inner dynein arms in trypanosomes remains unknown and needs further investigation. An interesting finding made in this report is the interdependence of TbCentrin3 and TbIAD5-1 for their stable assembly in the flagellum ( Figs 5 and 6 ), which appears to suggest that formation of the TbCentrin3–TbIAD5-1 complex is crucial for maintaining the stability of both proteins. Similar phenomenon was also observed in the TbKIN-C-TbKIN-D kinesin complex in which depletion of one kinesin unambiguously caused destabilization of its partner [25] , [26] , [27] . Notably, when the TbCentrin3–TbIAD5-1 complex is destabilized, both proteins were shifted from the flagellar fraction to cytosolic fraction and were degraded ( Figs 5d and 6c ). Intriguingly, when the outer-arm dynein complex was destabilized, shifting of an outer-arm dynein from the flagellar fraction to cytosolic fraction was also observed in trypanosomes [28] , suggesting similar assembly mechanisms for both the inner dynein arm and outer dynein arm in trypanosomes. Our results probably discovered a polar assembly process of the inner dynein arm at the distal tip of the growing flagellum, which was supported by the fact that depletion of TbCentrin3 caused gradual depletion of TbIAD5-1 from the distal tip of the new flagellum ( Fig. 5a and Supplementary Fig. 2 ). Such an assembly pattern is reminiscent of the polar assembly of the PFR in trypanosome flagellum [29] , [30] . It should be noted that similar patterns have been demonstrated for some components of the axoneme in Chlamydomonas previously, including the radial spoke protein 3 (ref. 31 ) and an inner dynein arm light chain protein p28 (ref. 32 ). Therefore, assembly of axonemal components in the flagellated organisms is likely to share the same mechanism. The precise mechanism by which centrin regulates the inner-arm dynein heavy chain and, hence, flagellar and ciliary motility in Chlamydomonas and Tetrahymena remains elusive. Genetic and molecular evidence for the implication of centrin in flagellar and ciliary motility in these two organisms is still lacking. As flagella and cilia respond to calcium by altering the beating pattern [33] and both the inner dynein arms and the radial spokes contain calcium-binding proteins, that is, centrins in the inner dynein arms and calmodulins in the radial spokes [33] , centrin may contribute to flagellar beating by binding to calcium via its conserved calcium-binding motifs, thereby enhancing the microtubule sliding velocity of the inner-arm dynein as observed in Tetrahymena [6] . Similar to the axoneme of the motile flagellum in other eukaryotes, the axoneme in trypanosome flagellum is also composed of nine outer doublet microtubules in a ring surrounding a central pair of singlet microtubules. The radial spokes extend from the outer doublet towards the central pair of microtubules and are linked to the inner dynein arms through a complex of proteins called the dynein regulatory complex [34] . In light of the conserved structure of the flagellar axoneme between trypanosomes and other flagellated eukaryotes, it is likely to be that the mechanisms of flagellar beating are also well conserved across different organisms. Indeed, both calmodulin and centrin were found in the flagellum of T. brucei . Calmodulin is mainly localized in the radial spokes and the PFR, but a low level of calmodulin was also detected at the central microtubule pair of the flagellar axoneme in trypanosomes [35] . RNAi of calmodulin resulted in defects in cell motility and total failure in PFR assembly in the procyclic form [36] . Our finding that TbCentrin3 RNAi caused depletion of TbIAD5-1 from the flagellum ( Fig. 5 ) suggests a crucial role of TbCentrin3 in maintaining the stability of this inner-arm dynein complex. Such a role of centrin may be well conserved in other flagellated and ciliated organisms, such as Chlamydomonas and Tetrahymena , where centrin is known to associate with the inner-arm dyneins. Trypanosome cell culture and RNAi Procyclic 29-13 cell line [37] was cultivated at 27 °C in SDM-79 medium containing 10% fetal bovine serum (Atlanta Biologicals, Inc.), 15 μg ml −1 G418 and 50 μg ml −1 hygromycin. Procyclic 427 strain was cultured at 27 °C in SDM-79 medium supplemented with 10% fetal bovine serum. RNAi of TbCentrin3 was carried out using the stem-loop RNAi construct. We modified the pLew100 vector [37] by introducing an Xho I and an Afl II site between the Hind III and BamH I sites, and we named this RNAi vector pSL for p S tem- L oop. Subsequently, a 500-bp fragment of human Plk1 gene was cloned between Xho I and Afl II sites. To make the stem-loop RNAi construct for TbCentrin3 RNAi, a 408-bp fragment corresponding to the N-terminal coding region of TbCentrin3 was amplified by PCR (forward primer: 5′-AAAATTCACAAGCTTAGTTGACGGACGCTCAGCGC-3′ and reverse primer: 5′-GAGTCATTGCTCGAGTTGACACACGATTGTCGTGG-3′) and cloned into the Hind III/ Xho I sites, and the same DNA fragment was amplified by PCR (forward primer: 5′-AAGGCCTCCCTTAAGTTGACACACGATTGTCGTGG-3′ and reverse primer: 5′-AAATGGGCAGGATCCAGTTGACGGACGCTCAGCGC-3′) and cloned into Afl II/ BamH I sites in an opposite direction. The resulting plasmid (pSL-TbCentrin3) was linearized by Not I digestion and electroporated into the 29-13 cell line. After 24 h, 2.5 μg ml −1 phleomycin was added to the culture medium. Transfectants were cloned by limiting dilution in a 96-well plate. For RNAi of TbIAD5-1, a 586-bp DNA fragment of TbIAD5-1 was amplified by PCR (forward primer: 5′-ATCTAGCCCCTCGAGAGTTGGTTGGCGACGATTAC-3′ and reverse primer: 5′-TTCGATATCAAGCTTAGGGACATTGCCGTACTGAC-3′) and cloned into the pZJM vector [38] , and transfection of 29-13 cells were carried out as above. To induce RNAi, the clonal cell line was incubated with 1.0 μg ml −1 tetracycline, and cell growth was monitored by counting the cell number with a haemacytometer. In situ epitope tagging of endogenous proteins The full-length coding sequence of TbCentrin3 was amplified by PCR (forward primer: 5′-TTG GGTACCGGGCCCATGGACGGAGATGATGGTTC-3′ and reverse primer: 5′-CTCACCAGCGGCCGCTTCTTAGGGGTGAGAAGC-3′) and cloned into the pC-EYFP-NEO vector, and the resulting construct was electroporated into the procyclic 427 cell line and the bloodstream 221 cell line. The same DNA fragment was also cloned into the pC-PTP-PAC vector and transfected into pSL-TbCentrin3 RNAi cell line and pZJM-TbIAD5-1 RNAi cell line, according to our published procedures [26] , [39] . Briefly, 10 7 cells were washed with 5 ml cytomix buffer (10 mM K 2 HPO 4 /KH 2 PO 4 , pH 7.6, 2 mM EGTA, pH 7.6, 120 mM KCl, 0.15 mM CaCl 2 , 25 mM Hepes, pH 7.6, 5 mM MgCl 2 , 0.5% Dextrose, 100 μg ml −1 BSA, 1 mM Hypoxanthine) and then resuspended in 0.4 ml cytomix buffer containing 20 μg plasmid DNA that has been linearized with appropriate restriction enzymes. Transfection of trypanosome cells was carried out in a BTX ECM 630 exponential decay wave electroporation system (Harvard Apparatus) with the following settings: 1,200 V, 25 Ω and 50 μF. After electroporation, cells were cultured in 10 ml fresh SDM-79 medium and incubated at 27 °C for 24 h. Stable transfectants were selected under 40 μg ml −1 G418 or 1 μg ml −1 puromycin, and clonal cell lines were obtained by limiting dilution on 96-well plates. Correct in situ tagging of one of the two TbCentrin3 alleles was confirmed by PCR and subsequent sequencing of the PCR fragment as well as western blotting with anti-GFP antibody (JL-8 clone, Clontech, 1:1,000 dilution) to detect TbCentrin3::EYFP fusion protein or anti-Protein A polyclonal antibody (Sigma-Aldrich, 1:5,000 dilution) to detect TbCentrin3::PTP fusion protein. Uncropped versions of blots are presented in Supplementary Figs 4–6 . DNA fragment corresponding to the C-terminal coding region of TbIAD5-1 was amplified by PCR (forward primer: 5′-GGCGAATTGGGTACCGGCTTGAGAGCATGTTCG-3′ and reverse primer: 5′-AGGATATTCCTTAAGATCATCTAGCATGCAGAG-3′) and cloned into the pC-3HA-PAC vector and transfected into the cell lines harbouring the pZJM-TbIAD5-1 RNAi construct, pSL-TbCentrin3 RNAi construct, or the pC-TbCentrin3-EYFP-NEO construct. DNA fragments corresponding to the C-terminal coding region of TbIAD5-2 and TbIAD3 were cloned into the pC-EYFP-PAC vector and transfected into the cell line harbouring the pSL-TbCentrin3 RNAi construct. Transfectants were selected with 1 μg ml −1 puromycin in addition to other appropriate antibiotics, and were cloned by limiting dilution. Motility analysis Sedimentation assay was performed according to the procedures published previously [40] . Briefly, the wild-type 29-13 cell line, the non-induced control cells, and TbCentrin3 RNAi cells and TbIAD5-1 RNAi cells after tetracycline induction for 3 days were each suspended to 5 × 10 6 cells per ml in fresh medium. Each cell line was cultured in two cuvettes and incubated at 27 °C. Optical density (600 nm) was measured every 2 h. When monitoring the OD 600 , one cuvette was resuspended for monitoring cell growth, whereas the other cuvette was not disturbed for monitoring sedimentation. The change in the OD 600 (ΔOD 600 ) was calculated by subtracting the OD 600 of the resuspended sample from that of the undisturbed sample according to published procedures [40] . The experiment was repeated three times. For motility tracing, the non-induced control cells, TbCentrin3 RNAi cells and TbIAD5-1 RNAi cells after tetracycline induction for 3 days were grown at ~5 × 10 6 cells per ml in culture medium and visualized at × 20 magnification under a light microscope. Images were captured every second for a total of 30 s using the Olympus IX81 automated inverted microscope equipped with a Hamamatsu Image EM EMCCD high-speed camera, and tracing of individual cell movement was monitored. For classification of runner, tumbler and immotile cells, we followed the criteria reported in previous publications [16] , [41] . Briefly, runner cells were classified as being able to move a long distance from one place to another. Tumbler cells still exhibited flagellar beating capability, but remained at the same location making circles or only moved a very small distance. Immotile cells were classified as cells that did not possess flagellar beating capability and did not move at all. For counting the runner, tumbler and immotile cells, cells were randomly chosen from the captured images and all cells in the images were counted. Preparation of cytoskeleton and flagellar skeleton Cytoskeleton preparation was performed according to previous procedures [42] , and preparation of flagellar skeleton was carried out according to published procedures [43] . Briefly, cells expressing TbCentrin3::EYFP were collected, washed three times with PBS and incubated in PEME buffer (0.1 M PIPES, pH 6.9, 2 mM EGTA, 1 mM MgSO 4 , 0.1 mM EDTA) containing 1% Nonidet P-40 at room temperature for 5 min. The resulting whole-cell lysate was then centrifuged to separate detergent-solubilized materials (S1) and pelleted cytoskeletons (P1). The cytoskeletons (P1) were either adhered onto coverslips and mounted in VectaShield mounting medium (Vector Labs) or washed in PMN buffer (10 mM Na 3 PO 4 , pH 7.4, 1 mM MgCl 2 , 150 mM NaCl) containing 1% Nonidet P-40 and then incubated in the same buffer containing 500 mM NaCl on ice for 30 min to depolymerize subpellicular microtubules. The P1 fraction was then centrifuged to separate the supernatant (S2) and the flagellar skeleton pellet (P2). The flagellar skeletons (P2) were adhered onto coverslips, mounted in VectaShield mounting medium and examined under a fluorescence microscope. Immunofluorescence microscopy Cells were adhered to coverslips and then treated with PEME buffer containing 1% NP-40 for 5 min. The following antibodies were used: fluorescein isothiocyanate-conjugated anti-HA monoclonal antibody (Clone HA-7, 1:400 dilution), anti-HA monoclonal antibody (clone HA-7, 1:400 dilution) and anti-Protein A polyclonal antibody (1:400 dilution). All three antibodies were purchased from Sigma-Aldrich. Cells were incubated with primary antibodies at room temperature for 1 h and then washed three times with PBS containing 0.1% Triton X-100. For anti-HA and anti-Protein A staining, cells were then incubated with Cy3-conjugated anti-mouse IgG or fluorescein isothiocyanate-conjugated anti-rabbit IgG (Sigma-Aldrich, 1:400 dilution) at room temperature for 1 h. The slides were mounted in VectaShield mounting medium (Vector Labs) containing DAPI (4′,6-diamidino-2-phenylindole) and examined using an inverted microscope (Model IX71, Olympus) equipped with a cooled charge-coupled device camera (model Orca-ER, Hamamatsu) and a PlanApo N × 60 1.42 numerical aperture differential interference contrast (DIC) objective. Images were acquired and processed using the Slidebook5 software (Intelligent Imaging Innovations, Inc.). Tandem affinity purification The full-length coding sequence of TbCentrin3 was amplified by PCR (forward primer: 5′-TTGGGTACCGGGCCCATGGACGGAGATGATGGTTC-3′ and reverse primer: 5′-TCTTCCAGCGGCCGCTTCTTAGGGGTGAGAAGC-3′) and cloned into the pN-PTP-NEO vector [14] , and the resulting construct was linearized and electroporated into the 427 cell line for in situ tagging of one of the two TbCentrin3 alleles. Successful transfectants were selected under 40 μg ml −1 G418 and cloned by limiting dilution. Correct in situ tagging of one of the two alleles of TbCentrin3 gene was confirmed by PCR and subsequent sequencing. Expression of PTP::TbCentrin3 fusion protein was verified by western blotting with anti-Protein C antibody (Roche, 1:500 dilution). Tandem affinity purification was carried out according to our previous procedures [25] with modifications. Briefly, 2 l procyclic cells (5 × 10 6 cells per ml) expressing PTP-tagged TbCentrin3 were lysed by sonication. The crude cell lysate was cleared by centrifugation and then incubated with 200 μl IgG Sepharose beads at 4 °C for 2 h. After overnight incubation with TEV (Tobacco Etch Virus) protease (200 U, Promega, Madison, WI), the eluate was incubated with 200 μl anti-protein C beads at 4 °C for 2 h. Proteins were then eluted with EGTA/EDTA elution buffer. Proteins were further precipitated with StrataClean resin (Stratagene), separated on SDS–PAGE and stained with silver solution (Pierce). Protein bands were excised from the gel and analysed by LC-MS/MS for protein identification. In-gel tryptic digestion and LC-MS/MS analysis In-gel digestion of proteins was carried out according to our published procedures [25] . One hundred and sixty nanograms of trypsin (Promega) was used for each band and digestion was carried out at 37 °C for 4 h. Peptides were then extracted from gel pieces with 50 ml of 50% acetonitrile, 5% formic acid and dried using speedvac. Samples were then reconstituted in 2% acetonitrile with 0.1% formic acid and injected onto Thermo LTQ Orbitrap XL (Thermo-Fisher Scientific, Bremen, Germany). Samples in 2% (v/v) acetonitrile and 0.1% (v/v) formic acid were analysed on an LTQ Orbitrap XL (Thermo-Fisher Scientific) interfaced with an Eksigent nano-LC 2D plus ChipLC system (Eksigent Technologies, Dublin, CA). The sample was loaded onto a ChromXP C18-CL trap column (200 μm i.d. × 0.5 mm length, 3 μm particle size) at a flow rate of 3 μl min −1 . Reversed-phase C18 chromatographic separation of peptides was carried on a on a ChromXP C18-CL column (75 μm i.d × 10 cm length, 3 μm particle size) at 300 nl min −1 . The LTQ Orbitrap was operated in the data-dependent mode to simultaneously measure full-scan MS spectra in the Orbitrap and the five most intense ions in the LTQ by CID, respectively. In each cycle, MS1 was acquired at target value 1E6 with resolution R =100,000 ( m/z 400) followed by top five MS2 scan at target value 3E4. The mass spectrometric setting is as follows: spray voltage was 1.6 KV, charge state screening and rejection of singly charged ion were enabled. Ion selection thresholds were 8,000 for MS2, 35% normalized collision energy, activation Q was 0.25 and dynamic exclusion was employed for 30 s. Raw data files were processed and search using Thermo Proteome Discoverer software or the Mascot search engine. Protein search was against Tb927-Trypanasoma database version 4. The search conditions used peptide tolerance of 10 p.p.m. and MS/MS tolerance of 0.8 Da with the enzyme trypsin and two missed cleavages. Co-immunoprecipitation Procyclic cells expressing PTP::TbCentrin3 were transfected with the pC-TbIAD5-1::3HA-PAC vector to express TbIAD5-1::3HA from one of its endogenous loci. Successful transfectants were selected under 1 μg ml −1 puromycin in addition to 40 μg ml −1 G418. For IP, 1 × 10 7 double transfectant cells were incubated in 0.5 ml trypanosome IP buffer (25 mM Tris-HCl, pH 7.6, 100 mM NaCl, 1 mM dithiothreitol, 1% Nonidet P-40 and protease inhibitor cocktail) and lysed by thorough sonication. The lysate was then cleared by centrifugation at 14,000 r.p.m. for 15 min in a microcentrifuge, and the cleared lysate was incubated with 50 μl IgG Sepharose beads at 4 °C for 2 h. After six washes with the IP buffer, beads were re-suspended in 10% SDS and supernatant was mixed with SDS–PAGE loading buffer. The supernatant was separated on SDS–PAGE and probed with anti-HA antibody for detecting TbIAD5-1::3HA and anti-Protein A polyclonal antibody (Sigma-Aldrich) for detecting PTP::TbCentrin3, respectively. For reciprocal IP, cleared cell lysate was incubated with 20 μl EZview Red anti-HA agarose gel to precipitate TbIAD5-1::3HA. The immunoprecipitate was separated by SDS–PAGE and immunoblotted with anti-Protein A polyclonal antibody (Sigma-Aldrich, 1:5,000 dilution) to detect PTP::TbCentrin3 and subsequently with horseradish peroxidase (HRP)-conjugated anti-HA monoclonal antibody (clone HA-7, 1:5,000 dilution) to detect TbIAD5-1::3HA. TbIAD5-1 and TbCentrin3 stability assay TbCentrin3 RNAi cell line harbouring endogenously 3HA-tagged TbIAD5-1 and TbIAD5-1 RNAi cell line harbouring endogenously PTP-tagged TbCentrin3 were induced for RNAi with 1.0 μg ml −1 tetracycline for 72 h. For MG-132 treatment, 64 h after RNAi induction 50 μg ml −1 MG-132 was added to the RNAi cells and incubated for an additional 8 h. Cells were harvested and total cell lysate was prepared by boiling for 5 min. Western blotting was carried out with HRP-conjugated anti-HA mAb (clone HA-7, Sigma-Aldrich, 1:5,000 dilution) or anti-Protein A pAb (Sigma-Aldrich, 1:5,000 dilution) to detect TbIAD5-1::3HA or TbCentrin3::PTP, respectively. The same blots were re-probed with anti-TbPSA6 (1:1,000 dilution), which detects the α6 subunit of the 26S proteasome [44] , for loading control. To prepare cytosolic and cytoskeletal fractions for western blotting, non-induced, RNAi-induced and RNAi-induced plus MG-132-treated cells were treated with PEME plus 1% NP-40 for 5 min and then centrifugated to separate cytosolic (S) and cytoskeletal (P) fractions. Western blotting was carried out with HRP-conjugated anti-HA monoclonal antibody (Clone HA-7, Sigma-Aldrich, 1:5,000 dilution) or anti-Protein A polyclonal antibody (Sigma-Aldrich, 1:5,000 dilution). The same blots were re-probed with anti-TbPSA6 (1:1,000 dilution) and anti-tubulin antibody (Sigma-Aldrich, 1:2,000 dilution) to detect cytosolic TbPSA6 protein and cytoskeletal tubulins, respectively. Protein band intensity was quantified with ImageJ software and normalized with the loading control. Transmission electron microscopy Cells were first fixed in glutaraldehyde, then treated with Millonig’s buffer for 10 min and finally incubated with 2% OsO 4 for 60 min at 4 °C. Cells were subsequently dehydrated by treating with 50% ethanol for 5 min, 70% ethanol for 10 min, 95% ethanol for 10 min and 100% ethanol for 10 min for three times. After dehydration, cells were embedded in resin by treating two times with 100% propylene oxide for 15 min, 50% LX-112 resin/50% propylene oxide for 2 h and finally with 100% LX-112 resin for 2 h. The fixed cells were embeded in BEEM capsules and then polymerized at 70 °C overnight. The 120-nm thin sections were cut using a Leica Ultracut-R microtome and a diamond knife (Daitome-US), placed on 150-mesh copper grids (Electron Microscopy Sciences, Hatfield, PA) and stained with 2% uranyl acetate for 15 min. The thin sections were then rinsed with water and incubated with Reynold’s lead citrate for 5 min. Grids were imaged using a JEOL 1400 TEM at 60 kv and captured with a Gatan charge-coupled device camera. How to cite this article: Wei, Y. et al . Centrin3 in trypanosomes maintains the stability of a flagellar inner-arm dynein for cell motility. Nat. Commun. 5:4060 doi: 10.1038/ncomms5060 (2014).